Phloem iron remodels root development in response to ammonium as the major nitrogen source 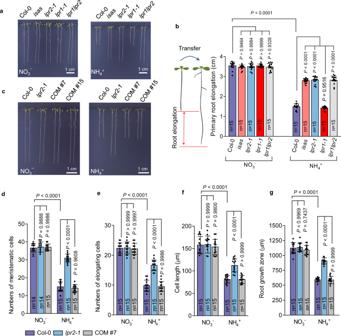Fig. 1: LPR2-dependent growth inhibition of primary roots in NH4+ medium. aPhenotype comparison of Col-0 and theisas,lpr2-1,lpr1-1, andlpr1lpr2mutants.bElongation of primary roots.cPhenotype comparison of Col-0,lpr2-1, and complementation lines (COM #7 and COM #15).dNumber of meristematic cells.eNumber of elongation cells.fLength of the first differentiated cell.gLength of the root growth zone (elongation plus meristem zone).b,d-gData shown are mean ± SD.Pvalues < 0.05 indicate significant differences (two-way ANOVA with post-hoc Tukey HSD test;n= number of seedlings). Four-day-old seedlings of the indicated genotypes were transferred to NO3−or NH4+medium with 100 µM Fe and analyzed 4 days after seedling transfer. Each experiment was repeated independently at least three times with similar results, and a representative experiment is shown. Plants use nitrate and ammonium as major nitrogen (N) sources, each affecting root development through different mechanisms. However, the exact signaling pathways involved in root development are poorly understood. Here, we show that, in Arabidopsis thaliana , either disruption of the cell wall-localized ferroxidase LPR2 or a decrease in iron supplementation efficiently alleviates the growth inhibition of primary roots in response to NH 4 + as the N source. Further study revealed that, compared with nitrate, ammonium led to excess iron accumulation in the apoplast of phloem in an LPR2-dependent manner. Such an aberrant iron accumulation subsequently causes massive callose deposition in the phloem from a resulting burst of reactive oxygen species, which impairs the function of the phloem. Therefore, ammonium attenuates primary root development by insufficiently allocating sucrose to the growth zone. Our results link phloem iron to root morphology in response to environmental cues. Nitrogen (N) is the essential nutrient required in the greatest quantity by plants. It is primarily acquired by plant roots in the forms of ammonium (NH 4 + ) and nitrate (NO 3 − ). Nevertheless, NH 4 + is notoriously toxic to most plants when present as the only or predominant N source [1] , which is not the case for NO 3 − . In fact, NH 4 + stress is of major importance to the ecology of soils that exhibit higher ammonification than nitrification rates, such as those found in wetlands, including saltmarshes, bogs, mangroves, and fens [2] , [3] , [4] . In addition, because of highly intensive tillage or waterlogged cultivation methods, many crop plants also suffer long-term NH 4 + stress induced by the over-application of N fertilizers [5] . Identification of the mechanisms underlying toxicity and detoxification of NH 4 + in plants is crucial for improving the adaptation of the plants in the presence of NH 4 + as the primary N source. Similar to many other abiotic cues, NH 4 + stress also inhibits the growth of primary roots (PRs); hence, stunted PR growth is recognized as a typical symptom of NH 4 + toxicity [6] , [7] . The uptake of NH 4 + by roots is the first step affecting cellular NH 4 + concentration and therefore is an important process affecting NH 4 + stress in plants. Knocking out NH 4 + transporters (AMTs) AtAMT1;1, AtAMT1;2, and AtAMT1;3 results in a 90% reduction in NH 4 + uptake and substantially decreases NH 4 + sensitivity [8] . The protein kinase AtCIPK23 phosphorylates and inactivates AtAMT1;1 and AtAMT1;2, and thus activation of AtCIPK23 expression by transcription factor AtSTOP1 has been identified as a mechanism for NH 4 + tolerance [9] , [10] . A decrease in NH 4 + uptake due to enhanced proton extrusion from the resulting activation of H + -ATPase has also been shown to be a mechanism for NH 4 + tolerance [11] , [12] . A high concentration of cellular NH 4 + also causes a variety of physiological damage in plants, such as disordered pH regulation, excess energy consumption, deficiency of mineral cations, increased oxidative stress, and disruption of hormonal homeostasis [4] , [6] , [13] . Lines of evidence have linked some of these effects to NH 4 + toxicity. For example, the reaction of the glutamine synthetase GLN2 in shoots over-produces protons, resulting in pH disorder and consequently contributing to NH 4 + toxicity in the shoots [14] ; NH 4 + stress results in excessive production of hormone ethylene, while EIN2- and EIN3-mediated ethylene signaling partly causes NH 4 + toxicity in shoots [15] , [16] . However, these physiological effects are indirectly related, and most of them explain NH 4 + toxicity in shoots but not in the roots [6] . Currently, only a few signaling events have been proposed to mediate NH 4 + -induced PR growth inhibition. A previous study showed that knockout of VTC1 , which encodes a GDP-mannose pyrophosphorylase, results in greater inhibition of PR growth under NH 4 + stress, but the underlying mechanism remains unclear [17] . Auxin was also suggested to be associated with the NH 4 + -sensitive phenotype of PRs [18] . However, it has been shown that the PR growth of auxin transport mutant aux1 is similar to that of the wild-type plant under NH 4 + stress [19] , leaving it open as to whether auxin plays a role in NH 4 + -induced PR growth inhibition. Therefore, the mechanisms, particularly the molecular pathways, underlying the negative impacts of NH 4 + in PR growth remain largely unknown [4] , [6] . In this work, we screened an Arabidopsis ( Arabidopsis thaliana ) transfer DNA (T-DNA) insertion mutant whose PR growth is insensitive to NH 4 + stress. The T-DNA insertion in this mutant was annotated in the gene LOW PHOSPHATE ROOT 2 ( LPR2 ), which encodes a ferroxidase. Since the biological processes of roots might be artificially affected by photo-Fenton reactions resulting from the light-irradiated rooting conditions [20] , [21] , a shaded rooting system was used in our study. We further identified a mechanism that connects remodeling of root development to NH 4 + stress: the NH 4 + induces massive Fe accumulation in phloem via the action of LPR2, and as a result, arrests PR development due to the inhibition of phloem function. The NH 4 + -sensitive phenotype of PRs depends on the action of LPR2 An NH 4 + -insensitive Arabidopsis mutant isas was initially screened from a T-DNA insertion library [22] using transparent Petri dishes with a light-irradiated rooting medium. This mutant was found to be the SALK_056696 line, with the T-DNA insertion in the second exon of LPR2 (AT1G71040) (Supplementary Fig. 1a, b ). qRT-PCR and immunoblot assay showed that isas is most probably a LPR2 knockout mutant (Supplementary Fig. 1c, d ). As natural soils normally have pH-buffering capacity, the pH buffer MES was added to the growth media in our study, unless specified otherwise. When grown on a control medium with NO 3 − as the N source, the isas roots did not differ morphologically from wild-type Col-0 roots. In the medium with NH 4 + as the N source, however, the isas mutants showed better PR growth than Col-0 seedlings did (Supplementary Fig. 2 ). Unless specified otherwise, we used a black plastic sheet to cover the roots to exclude light irradiation in the remaining studies (Supplementary Fig. 3 ). Under such root-shaded conditions, the isas mutants still had greater PR elongation in the NH 4 + -N source than Col-0 seedlings did (Fig. 1a, b ). In addition, another T-DNA insertion mutant, lpr2-1 (SALK_091930) [23] , which is also probably a knockout mutant (Supplementary Fig. 1 ), had a similar NH 4 + -insensitive phenotype. The NH 4 + sensitivities of both lpr2 mutants were also examined in unbuffered conditions, and both mutants consistently had better PR growth than Col-0 seedlings did in the NH 4 + -N source without MES (Supplementary Fig. 4 ). These results show that the inhibitory effect of NH 4 + on PR growth could be uncoupled by disruption of LPR2. Fig. 1: LPR2-dependent growth inhibition of primary roots in NH4+ medium. a Phenotype comparison of Col-0 and the isas , lpr2-1 , lpr1-1 , and lpr1lpr2 mutants. b Elongation of primary roots. c Phenotype comparison of Col-0, lpr2-1 , and complementation lines (COM #7 and COM #15). d Number of meristematic cells. e Number of elongation cells. f Length of the first differentiated cell. g Length of the root growth zone (elongation plus meristem zone). b , d - g Data shown are mean ± SD. P values < 0.05 indicate significant differences (two-way ANOVA with post-hoc Tukey HSD test; n = number of seedlings). Four-day-old seedlings of the indicated genotypes were transferred to NO 3 − or NH 4 + medium with 100 µM Fe and analyzed 4 days after seedling transfer. Each experiment was repeated independently at least three times with similar results, and a representative experiment is shown. Full size image LPR1 (AT1G23010) is a close paralog of LPR2 [23] . However, the NH 4 + -sensitive PR phenotype of the lpr1-1 mutant did not differ from that of Col-0 seedlings (Fig. 1a, b ). Moreover, the lpr1lpr2 double mutants did not have greater insensitivity to NH 4 + than lpr2 single mutants did. Accordingly, the NH 4 + sensitivity of PRs was only associated with LPR2 and not with LPR1 . We also generated pLPR2::LPR2-YFP transformants in the lpr2-1 background. These complementation lines (COM#7 and COM#15) had moderately higher LPR2 expression and LPR2 abundance than Col-0 seedlings did (Supplementary Fig. 5 ) and fully restored the inhibitory effect of NH 4 + on PR growth (Fig. 1c ). These results further demonstrate that LPR2 is responsible for the NH 4 + sensitivity of PRs. Root elongation is controlled by cell division and differentiation along the longitudinal axis of the root [24] . Here, we showed that the meristematic cell numbers in PRs of Col-0 and COM#7 seedlings in the NH 4 + -N source were both decreased by ~60% compared with those in the NO 3 − -N source, whereas only a slight decrease was observed in lpr2-1 mutants (Fig. 1d ). This indicates that LPR2 acts to accelerate a shift from cell division to differentiation. In addition, both the elongation cell number and the first differentiated cell length in PRs of Col-0 and COM#7 seedlings were also greatly reduced by NH 4 + , and such reductions were clearly diminished in the lpr2-1 PRs (Fig. 1e, f ). As a result, in the NH 4 + , the lpr2-1 mutants had less growth stunting in the root growth zone (meristem plus elongation zone) than Col-0 and COM#7 seedlings did (Fig. 1g ). Therefore, the PR growth inhibition resulting from NH 4 + stress highly depends on LPR2 and is initiated by an accelerated shift from cell division to differentiation in the meristem zone, followed by early differentiation of elongating cells. LPR2 encodes a cell wall ferroxidase and is irreplaceable by LPR1 Prediction by the SignalP 5.0 algorithm [25] showed that both LPR1 and LPR2 contained a putative secretory signal peptide at the N-terminal region (Supplementary Fig. 6 ). Consistent with this prediction, confocal analysis of p35S::LPR2-GFP transformants revealed that LPR2-GFP fluorescence mainly resided in the cell wall matrix (Fig. 2a, b ), which is very similar to the subcellular localization of LPR1 [26] . LPR1 was previously characterized to have ferroxidase activity that converts Fe 2+ to Fe 3+, [26] , [27] . As expected, the recombinant GST-LPR2 protein from Escherichia coli also had obvious ferroxidase activity, and exhibited a typical Michaelis–Menten kinetic with a K m and V max of 17.43 µM and 22.10 µM/min/mg protein, respectively (Fig. 2c, d ). Fig. 2: LPR2 is a cell wall ferroxidase and is irreplaceable by LPR1. a Fluorescence co-localization of LPR2-GFP and propidium iodide in cells of p35S::LPR2-GFP roots. b Fluorescence of LPR2-GFP and FM4-64 in cells of p35S::LPR2-GFP roots after plasmolysis with 0.8 M sorbitol. Four-day-old seedlings were transferred to NH 4 + medium with 100 µM Fe, and confocal analyses were performed 4 days after seedling transfer. c Ferroxidase activities of recombinant GST-LPR2. Ferroxidase assay using 1 μg purified GST-LPR2 protein. Pink indicates the Fe 2+ -ferrozine complex. The substrate Fe 2+ was added in the form of Fe(NH 4 ) 2 (SO 4 ) 2 ·6H 2 O at an initial concentration of 50 μM. d Fe 2+ concentration-dependent (0–300 μM) ferroxidase activity of GST-LPR2 protein. Data shown are mean ± SD of three biological replicates. e , f Phenotype of lpr2-1 mutant lines with LPR2 promoter-confined tissue-specific expression of LPR1 CDS and LPR1 genomic . Four-day-old seedlings of the indicated genotypes were transferred to NO 3 − or NH 4 + medium with 100 µM Fe and analyzed 4 days after seedling transfer. Two ( c , d ) or three ( a , b , e , f ) independent experiments were performed with similar results, and one representative experiment is shown. Full size image Considering the similarities of LPR2 and LPR1 in both subcellular localization and enzymatic reaction, we explored whether the role of LPR2 in mediating NH 4 + sensitivity could be filled by LPR1. We used the LPR2 promoter to confine the site of LPR1 expression in the lpr2-1 mutant. However, although both pLPR2::LPR1 CDS / lpr2-1 and pLPR2::LPR1 genomic / lpr2-1 transformants had comparable or slightly higher expression levels of LPR1 compared with that of LPR2 in Col-0 seedlings (Supplementary Fig. 7 ), they still showed similar PR growth as that of the lpr2-1 seedlings in the NH 4 + -N source (Fig. 2e, f ). Therefore, LPR2 is irreplaceable by LPR1 in mediating NH 4 + sensitivity, which may explain why only LPR2 and not LPR1 acts to suppress PR growth in the presence of NH 4 + . The LPR2-mediated NH 4 + -sensitive PR phenotype depends on the action of Fe We next asked how LPR2 mediates the NH 4 + sensitivity of PRs. Disruption of LPR2 did not affect the NH 4 + level in roots (Supplementary Fig. 8 ), showing that LPR2-mediated NH 4 + sensitivity is not associated with NH 4 + accumulation. Since LPR2 is a ferroxidase, the role of Fe in regulating NH 4 + sensitivity of PRs was investigated. We first grew Arabidopsis seedlings in media with different doses of Fe. Fe doses ≤10 µM ensured a similar PR growth of Col-0 between NH 4 + - and NO 3 − -N sources, whereas ≥50 µM induced a clear dose-dependent inhibition of PR growth in the NH 4 + -N source (Supplementary Fig. 9 and Fig. 3a ). In contrast, supplementing deferoxamine or ferrozine, two potent Fe chelators, almost completely rescued PR growth of Col-0 seedlings in the NH 4 + -N source with 100 µM Fe (Supplementary Fig. 10 ). The inhibitory effect of NH 4 + on root growth of rice plants was also uncoupled by lowering Fe supply (Supplementary Fig. 11 ). These results indicate that the NH 4 + sensitivity of roots strongly depends on the action of Fe. Given that Fe-free (0 µM) and high-Fe (≥200 µM) conditions may respectively cause Fe deficiency and Fe excess in Arabidopsis, we used 10 and 100 µM Fe, defined as low Fe (Fe low ) and sufficient Fe (Fe suff ), respectively, in the remaining evaluations. The difference in NH 4 + sensitivity between lpr2 mutants and either Col-0 or COM#7 seedlings was completely abolished when the Fe concentration was lowered from Fe suff to Fe low (Fig. 3b ), showing that the LPR2-mediated NH 4 + -sensitive phenotype depends on the action of Fe. Fig. 3: Fe-dependent inhibition of primary root growth in NH4+ medium. a Primary root elongation of Col-0 seedlings in NO 3 − -N or NH 4 + -N source with various doses of Fe. Center line represents mean and bounds of box are SD; whiskers indicate the minimum and maximum values; n = number of seedlings. P values <0.05 indicate significant interactions between N form and Fe dose (two-way ANOVA with post-hoc Tukey HSD test). b NH 4 + -sensitivity comparison of Col-0, isas , lpr2-1 , and complementation line COM#7 in Fe suff (100 µM) and Fe low (10 µM) conditions. c Fe deposition indicated by Perls/DAB staining in primary roots. d Close-up view of Fe deposition in root stele of Col-0 seedlings grown in Fe suff NH 4 + medium. Ep epidermis, Co cortex, En endodermis, Pe pericycle, Ph phloem, Xy xylem. e Perls/DAB staining in the phloem of the primary roots of Col-0 seedlings grown in Fe suff NH 4 + medium. Red and green arrows show Fe depositions at lateral cell walls and sieve plates of the phloem, respectively. f Acetone washed-Perls/DAB staining in phloem of the primary roots of Col-0 seedlings grown in Fe suff NH 4 + medium. The Perls/DAB-stained roots were washed with acetone for 3 h. Four-day-old seedlings of the indicated genotypes were transferred to NO 3 − or NH 4 + medium with various doses of Fe supply and analyzed 4 days after seedling transfer. Each experiment was repeated independently three times with similar results, and a representative experiment is shown. Full size image Furthermore, we tested whether Fe plays a role in NH 4 + sensitivity of PRs when the N source has a high NH 4 + /NO 3 − ratio (10:2). Similarly, the difference in PR growth inhibition between lpr2 mutants and Col-0 seedlings at a high NH 4 + /NO 3 − ratio was also abolished by lowering Fe supplement (Supplementary Fig. 12 ). Therefore, Fe is required for the remolding of PR development when NH 4 + is the only or predominant N source. NH 4 + induces Fe deposition in the phloem The strong dependence of the NH 4 + -sensitive PR phenotype on Fe raised the question of whether NH 4 + stress affects Fe deposition in roots. We used an Fe-specific histochemical procedure, Perls/3,3’-diaminobenzidine (DAB) staining [28] , to visualize Fe distribution in PRs. For Col-0 and lpr1-1 seedlings with Fe suff , the NH 4 + -N source resulted in massive Fe deposition in root stele compared to that of the NO 3 − -N source (Fig. 3c and Supplementary Fig. 13a ). In contrast, the NH 4 + -induced Fe deposition was completely abolished by either disruption of LPR2 in lpr2-1 mutants or Fe low treatment in Col-0 seedlings. The complementation line COM#7 restored the Fe deposition in root stele in the NH 4 + -N source with Fe suff . These results indicate that NH 4 + -induced Fe deposition in root stele depends on LPR2 as well as on a sufficient Fe supply. Notably, these respective Fe depositions across the various genotypes and Fe-dose treatments were negatively correlated with PR growth in the NH 4 + -N source (Fig. 3b ), suggesting that the Fe deposition in root stele determines the PR growth response to NH 4 + stress. Surprisingly, in the presence of either NO 3 − or NH 4 + , Fe low treatment resulted in a higher Fe deposition in the root stem cell niche (SCN) of Col-0, lpr2-1 , and COM#7 seedlings compared with that with Fe suff treatment (Fig. 3c ). Nevertheless, although no Fe deposition was detected in the SCN of lpr1lpr2 seedlings (Supplementary Fig. 13b ), this double mutant displayed similar NH 4 + insensitivity as that of the lpr2-1 mutant (Fig. 1c ), indicating that the NH 4 + sensitivity of PRs is independent of the Fe deposition in SCN. A close-up view of Perls/DAB-stained Col-0 roots from Fe suff NH 4 + treatment showed that the greatest Fe deposition was in phloem cells (Fig. 3d ). At higher magnification, Fe was found to be mainly located at the periphery of sieve elements (Fig. 3e ). This periphery is probably the apoplast of phloem, because the LPR2 responsible for this Fe deposition is a cell wall-resident protein. Since the phloem vasculature was difficult to plasmolyze using the methods of osmotic dehydration, we used acetone to wash off the plasmalemma. This procedure did not alter Fe deposition at the periphery of sieve elements (Fig. 3f ), providing further support for apoplastic Fe deposition in the phloem. Unexpectedly, the NH 4 + -N source with Fe suff resulted in heavy Fe deposition in all cell types of Col-0 PRs under light-irradiated rooting conditions, which was significantly different from that observed under root-shaded conditions (Supplementary Fig. 14 ). The result strongly suggests that the impact of artificial light irradiation on roots cannot be neglected in studying the mechanisms of root growth responses to NH 4 + , even though root growth inhibition by NH 4 + is barely affected by the light irradiation on roots. LPR2 distributes in root stele and is upregulated by NH 4 + The NH 4 + -induced phloem-specific Fe deposition prompted us to analyze the tissue distribution of LPR2 in PRs of pLPR2::LPR2-YFP/lpr2-1 transformants. LPR2-YFP was mainly distributed in the root stele, but its abundance was lower in the NO 3 − -N source. LPR2-YFP fluorescence was increased in the NH 4 + -N source, while the dose of Fe had little effect on this response (Fig. 4a ). Unexpectedly, LPR2 was found to be ubiquitously distributed in the whole root stele except in the xylem (Fig. 4b ), an area much larger than the Fe deposition region (i.e., phloem). This suggests that other factor(s) are required for phloem-specific Fe deposition and NH 4 + -induced PR growth inhibition. Unfortunately, we were unable to identify the relative factor(s) in the present study. Fig. 4: Distribution of LPR2 in roots and its response to NH4+. a pLPR2::LPR2-YFP expression in primary roots of complementation line COM#7. Roots were counterstained with propidium iodide (purple fluorescence) and analyzed for YFP fluorescence (green). b Radial section (top) and close-up view (bottom) of pLPR2::LPR2-YFP expression in a root of a COM#7 seedling grown in Fe suff NH 4 + medium. c LPR2 expression in Col-0 roots. Relative expression levels were normalized to the geometric mean of expression of UBQ10 and EF1α . d , e Representative gels and relative protein levels in Col-0 roots. Relative LPR2 levels were estimated from the ratio of the signal intensity of LPR2 to that of actin from the same sample. c , e Data shown are mean ± SD of three biological replicates. P values < 0.05 indicate significant differences (two-way ANOVA with post-hoc Tukey HSD test). Four-day-old seedlings of the indicated genotypes were transferred to NO 3 − or NH 4 + medium with Fe suff (100 µM) or Fe low (10 µM) and analyzed 4 days after seedling transfer. Each experiment was repeated independently three times with similar results, and a representative experiment is shown. Full size image LPR1 distribution in PRs was also examined in pLPR1::LPR1-YFP / lpr1-1 transformants. The abundance of LPR1-YFP was lower in the presence of either N source, but it was mainly distributed in the SCN of the root apical meristem and slightly expanded to endodermal cell layers (Supplementary Fig. 15 ). The difference in tissue distribution may be another part of the explanation of why LPR1 does not play a role in mediating the NH 4 + -sensitive phenotype as LPR2 does. The response of LPR2 in Col-0 roots to NH 4 + was also examined. Consistent with the above confocal result, either the LPR2 expression or the LPR2 abundance in Col-0 roots showed an increase under NH 4 + relative to that under NO 3 − , which was also irrespective of the Fe supplementation dose (Fig. 4c–e ). Therefore, NH 4 + rather than Fe upregulates LPR2. Interestingly, although the LPR2 expression in p35S::LPR2-GFP overexpression lines was similar between two N sources, the LPR2-GFP abundance in the NH 4 + -N source was higher than that in the NO 3 − -N source (Supplementary Fig. 16 ), indicating a post-transcriptional regulation for LPR2. It is worth noting that, although LPR2 was slightly overexpressed in pLPR2::LPR2-YFP/lpr2-1 complementation lines (Supplementary Fig. 5 ), their PRs had a similar NH 4 + -sensitive phenotype as that of Col-0 seedlings (Fig. 1d ). Furthermore, the PRs of p35S::LPR2-GFP overexpression lines also had a similar NH 4 + sensitivity as that of Col-0 PRs (Supplementary Fig. 17a ). These results indicate that the upregulated portion of LPR2 makes little contribution to NH 4 + sensitivity and further support that, although LPR2 is essential, additional factor(s) are also required for NH 4 + -induced PR growth inhibition. It is worth noting that the p35S::LPR2-GFP overexpression lines showed irregular Fe deposition in PRs in the NH 4 + -N source (Supplementary Fig. 17b ), indicating that NH 4 + -induced phloem-specific Fe deposition depends on the stele-specific distribution of LPR2. NH 4 + -induced Fe deposition triggers a burst of reactive oxygen species (ROS) To understand how LPR2-mediated Fe deposition inhibits PR growth in the NH 4 + -N source, we performed a whole transcriptome sequencing (RNA-seq) analysis of gene expression in the roots of Col-0 and lpr2-1 seedlings (Supplementary Data 1a ). The reliability of RNA-seq data was confirmed by qRT-PCR assay for the expression of ten randomly selected genes with different abundances (Supplementary Fig. 18 ). As Fe low treatment and LPR2 disruption similarly alleviated PR growth inhibition in the NH 4 + -N source, we screened differentially expressed genes (DEGs) (−1 > log 2 [fold change] > 1; P value <0.05) by performing pairwise comparisons of transcript abundances either between the two Fe treatments or between lpr2-1 and Col-0 with Fe suff treatment (Supplementary Data 1b–e ). In the NO 3 − -N source, there were only 11 DEGs between the two Fe treatments for Col-0 seedlings and 87 DEGs between the two genotypes that received Fe suff treatment (Supplementary Fig. 19a, b ). These DEGs are unlikely related to PR development because either Fe low treatment or LPR2 disruption had little effect on PR growth in NO 3 − -N source. We subsequently focused on DEGs in the NH 4 + -N source. There were 182 DEGs (101 upregulated; 81 downregulated) between two Fe treatments for Col-0 seedlings and 130 DEGs (58 upregulated; 72 downregulated) between two genotypes that received Fe suff treatment (Fig. 5a and Supplementary Fig. 19c, d ). In these two comparisons, however, we did not find any DEGs currently known to be related to NH 4 + toxicity (Supplementary Data 1f ). Interestingly, the ratio of overlapped DEGs in the above two comparisons was high (Fig. 5a ), and Gene Ontology (GO) enrichment analysis showed that the biggest cluster in both comparisons was related to “response to oxidative stress” (Fig. 5b ). Fig. 5: Fe-dependent primary root growth inhibition by NH4+ is associated with a burst in reactive oxygen species (ROS). a , b Venn diagram and Gene Ontology enrichment analysis of differentially expressed genes (DEGs) that are up- and downregulated in the pairwise comparisons of Col-0 Fe low vs. Col-0 Fe suff and lpr2-1 Fe suff vs. Col-0 Fe suff in the NH 4 + -N source. The size of the circle represents gene numbers, and the color represents the value of P -adjust the was calculated by hypergeometric tests and adjusted for multiple testing using FDR. RNA sequencing was conducted with three biological replicates per line and condition. c ROS visualization in primary roots of Col-0, lpr2-1 , and complementation line COM#7 seedlings by H 2 DCFDA staining. d Close-up view of H 2 DCFDA staining in primary roots of Col-0 seedlings grown in Fe suff NH 4 + medium. e Co-localization of false color representation of H 2 O 2 and fluorescence of phloem marker esculin in primary roots of roGFP2-Orp1 seedlings grown in Fe suff NH 4 + medium. f , g Dose-response relationship of the primary root elongation of Col-0 seedlings plotted as a function of the concentration of ROS scavengers. Data shown are mean ± SD. n = number of seedlings. P values < 0.05 indicate significant differences (one-way ANOVA with post-hoc Tukey HSD test). h Images of the effects of 750 µM dimethyl thiourea (DMTU) and 200 µM 4-hydroxy-TEMPO (TEMPO) on Col-0 seedlings. Four-day-old seedlings of the indicated genotypes were transferred to NO 3 − or NH 4 + medium with Fe suff (100 µM) or Fe low (10 µM) with or without the indicated ROS scavengers. Analyses were performed 4 days after seedling transfer. The experiments ( c – h ) were repeated independently three times with similar results, and representative data from one experiment are shown. Full size image The above results prompted us to monitor ROS formation in roots. We first histologically visualized ROS using 2’,7’-dichlorodihydrofluorescein diacetate (H 2 DCFDA), a fluorescent ROS indicator. The data showed that NH 4 + resulted in clear ROS formation in root stele, which depended on either LPR2 action or sufficient Fe supplementation (Fig. 5c ). The ratiometric fluorescent reporter protein roGFP2-Orp1 was recently shown to report the level of intracellular H 2 O 2 [29] . Because of the passage of extracellular H 2 O 2 across the plasma membrane via aquaporins [30] , [31] , the extracellular H 2 O 2 formation can also be indirectly reflected by roGFP2-Orp1 reporter in its neighboring cells [29] . Consistent with the observed ROS formation, the roGFP2-Orp1 reporter showed that NH 4 + also triggered a burst of H 2 O 2 in root stele under Fe suff conditions (Supplementary Fig. 20 ). A close-up view of H 2 DCFDA-stained roots revealed that the NH 4 + -triggered burst of ROS mainly occurred in the phloem (Fig. 5d ) and resembled the pattern of NH 4 + -induced Fe deposition. This finding was further supported by the roGFP2-Orp1 reporter in that the NH 4 + -induced H 2 O 2 accumulation was overlaid well with the phloem marker esculin (Fig. 5e ). ROS act downstream of Fe deposition to mediate growth response to NH 4 + The above results implied that the remodeling of root development in response to NH 4 + stress may be associated with a burst of ROS. Therefore, ROS scavengers were used to test this assumption. Unexpectedly, the addition of either ascorbic acid (ASA) or glutathione (GSH) to the NH 4 + medium with Fe suff resulted in greater inhibition of PR growth. This is probably because either ASA or GSH can enhance the production of hydroxyl radicals (·OH)—one of the most deleterious ROS—under Fe-rich conditions by Fenton reactions [32] . We also tested the effect of the H 2 O 2 scavenger potassium iodide, but this compound showed high toxicity to plants in our growth condition because it could inhibit PR growth even in the NO 3 - medium. Thus, we used other milder ROS scavengers, including dimethyl thiourea (DMTU) and 4-hydroxy-TEMPO (TEMPO), to counteract excess ROS production. Application of either of these scavengers to Col-0 seedlings had little effect on the growth of PRs in NO 3 - medium with Fe suff (Supplementary Fig. 21 ) but significantly restored PR growth in NH 4 + medium with Fe suff in a dose-dependent manner (Fig. 5f–h ). The result suggests that Fe-dependent PR growth inhibition in NH 4 + -N source could be associated with excessive ROS formation. We also examined Fe deposition after DMTU and TEMPO treatments. Although the PR growth of Col-0 seedlings in Fe suff NH 4 + medium was restored in the presence of ROS scavengers, Fe deposition in root phloem was still observed (Supplementary Fig. 22 ). Therefore, ROS very likely act downstream of Fe deposition to remodel root development in the NH 4 + -N source. However, application of either ROS scavenger lengthened the distance between the starting site of NH 4 + -induced Fe deposition and the root tip. This is probably associated with improved development of the root growth zone owing to ROS scavengers. NH 4 + induces callose deposition in the phloem There is growing evidence that ROS regulates callose deposition [33] . We, therefore, examined callose formation by aniline blue staining (Fig. 6a ). For Fe suff -treated Col-0 seedlings, the NH 4 + -N source resulted in massive callose deposition in root stele relative to that with the NO 3 − -N source. This NH 4 + -induced callose deposition was completely inhibited by either disruption of LPR2 in lpr2-1 seedlings or Fe low treatment in Col-0 seedlings. The complementation line COM#7 behaved similarly to Col-0. Therefore, NH 4 + induces callose deposition in root stele in LPR2- and Fe-dependent manners. Furthermore, both the close-up and the radial section views of the Fe suff NH 4 + Col-0 roots showed that callose deposition was mainly localized in two poles of the root stele (Fig. 6b ). Fig. 6: Fe-dependent callose deposition in the phloem via reactive oxygen species (ROS) in response to NH4+. a Callose detection in primary roots of Col-0, lpr2-1 , and complementation line COM#7 seedlings by aniline blue staining. b Radial section (top) and close-up view (bottom) of aniline blue staining in primary roots of Col-0 seedlings grown in Fe suff NH 4 + medium. c Fluorescence co-localization of GFP-sporamin and aniline blue staining in pSUC2::GFP-sporamin roots. d ROS scavengers abolished the NH 4 + -induced callose deposition. Four-day-old seedlings of the indicated genotypes were transferred to NO 3 − or NH 4 + medium with Fe suff (100 µM) or Fe low (10 µM) with or without the indicated ROS scavenger. Each experiment was repeated independently three times with similar results, and a representative experiment is shown. Full size image To determine the cell type for these two poles, aniline blue staining was performed in roots of pSUC2::GFP-sporamin transformants in which the GFP-sporamin marker was restricted in the phloem files, including sieve elements and companion cells [34] . Confocal analysis revealed that the aniline blue staining overlaid well with the GFP-sporamin marker in the roots subjected to Fe suff NH 4 + treatment, showing that NH 4 + -dependent callose deposition is localized in the phloem (Fig. 6c ). At high magnification, callose was found to be located at the periphery of sieve elements (Supplementary Fig. 23 ), which is strikingly similar to the localization of the Fe deposition. It is worth noting that, although neither DMTU nor TEMPO abolished the NH 4 + -induced Fe deposition in the root phloem (Supplementary Fig. 22 ), they substantially blocked callose deposition in the phloem (Fig. 6d ). Therefore, the burst of ROS acts downstream of Fe deposition to induce callose deposition in response to NH 4 + stress. Impaired phloem action is responsible for the growth response to NH 4 + As callose deposition in the phloem may affect phloem action, the phloem-mobile probe esculin [35] was used to evaluate the impacts of NH 4 + stress on phloem action. The phloem transport velocity (PTV) was determined by dividing the distance of esculin traveled between two marks by the elapsed time [36] . The data showed that NH 4 + significantly inhibited the PTV in PRs of Col-0 seedlings compared with the NO 3 − -N source under Fe suff conditions, whereas either disruption of LPR2 in lpr2-1 mutants or Fe low treatment in Col-0 seedlings completely reversed this inhibition. The complementation line COM#7 behaved similarly to Col-0 (Fig. 7a ). We then focused on phloem unloading. Once the esculin was imported into the root tip, individual images were recorded along with their times of acquisition [37] . As expected, NH 4 + strongly arrested esculin unloading from phloem in the root growth zone in LPR2- and Fe-dependent manners (Fig. 7b ). These results demonstrate that NH 4 + impairs phloem function via the actions of LPR2 and Fe. Fig. 7: Inhibition of phloem action and sucrose complementation of primary root growth in NH4+ medium. a , b Phloem transport velocity and phloem unloading of esculin. Center line represents mean and bounds of box are SD; whiskers indicate the minimum and maximum values. P values < 0.05 indicate significant differences (two-way ANOVA with post-hoc Tukey HSD test, n = 12 seedlings per line and condition). Four-day-old seedlings of Col-0, lpr2-1 , and complementation line COM#7 were transferred to NO 3 − or NH 4 + medium with Fe suff (100 µM) or Fe low (10 µM) and analyzed 4 days after seedling transfer. c Growth response of detached primary roots to localized sucrose supply. Data shown are mean ± SD. P values < 0.05 indicate significant differences (two-way ANOVA with post-hoc Tukey HSD test, n = 16 detached primary roots per line and condition). Inset: Scheme depicting the growth response analyses of detached primary roots to localized sucrose supply. Roots (1 cm) were cut from four-day-old seedlings. The detached roots were then transferred to a vertical two-layer split agar system of either NO 3 − or NH 4 + medium with Fe suff or Fe low . The upper layers were treated with various doses of sucrose, and the lower layers were absent of sucrose. Analyses were performed 3 days after seedling transfer. Each experiment was repeated independently three times similar results, and a representative experiment is shown. Full size image As esculin is loaded into the phloem by the sucrose transporter SUC2 [35] , [38] , the impaired phloem transport and unloading of esculin reflect the inhibition of sucrose supply to the root growth zone. We, therefore, examined whether the LPR2-dependent NH 4 + -sensitive phenotype was associated with insufficient sucrose allocation to the root growth zone. Because all the above tests were performed using seedlings fed with 1% sucrose, we first needed to clarify an artificial effect from exogenous sucrose. The lpr2-1 mutants still exhibited better PR growth than Col-0 seedlings did in the sucrose-free NH 4 + medium, although the difference between them was slightly diminished compared with that in plants supplemented with 1% sucrose (Supplementary Fig. 24 ). Therefore, the genotype-specific growth response to the N source largely depends on the native biological processes of plants. In subsequent tests, we used detached PRs to eliminate the potential effects of the sucrose source of shoots from different genotypes on their root growth. The detached PRs were transferred to a vertical two-layer split agar system with sucrose absent in the lower layer and various doses of sucrose present in the upper layer (Fig. 7c ). In sucrose-free treatment, the detached PRs almost completely lost growth ability regardless of N source and genotype, indicating the importance of phloem-transported sucrose in maintaining root growth. For Col-0 seedlings, the growth difference of detached PRs between NO 3 − -N and NH 4 + -N sources with Fe suff highly depended on the dose of sucrose: the difference was the most significant with 1% sucrose treatment, but it was diminished with lower sucrose doses because PR growth was inhibited in both N sources. Notably, the inhibitory effect of NH 4 + on the growth of detached PRs of Col-0 seedlings was completely uncoupled by the elevation of sucrose to 3% or more. The detached PRs of lpr2-1 mutants showed similar growth between the two N sources in all sucrose treatments, probably because LPR2 disruption protected the phloem from impairment due to NH 4 + stress. The complementation line COM#7 behaved similarly to Col-0. Taken together, the above results point to a connection between the effect of NH 4 + -induced stress on root morphological response and insufficient sucrose allocation resulting from inhibited phloem action. NH 4 + can be directly assimilated after absorption into plant cells, whereas NO 3 − needs to be reduced to NH 4 + in an energy-consuming manner before it can be utilized by plants [39] , [40] . This raises a critically puzzling question because, although NH 4 + is a theoretically preferred N source for plants, it inhibits PR growth when it is the only or predominant N source. Our study provides insights into the related factors that contribute to the adjustment of PR development in response to NH 4 + stress by revealing the essential role of phloem Fe deposition in determining the NH 4 + -sensitive phenotype of PRs. Furthermore, increased external Fe availability intensifies NH 4 + -induced PR growth inhibition (Fig. 3a ). Therefore, the occurrence of NH 4 + toxicity in roots is not a single-factor event: Fe is also involved in this process. Notably, the conditions of soils that favor NH 4 + formation also favor Fe solubilization. For example, in wetlands with anoxic conditions, the levels of soluble Fe can easily exceed 10 mg kg −1 (~180 µmol kg −1 ) [41] , [42] ; in acidic soils rich in NH 4 + due to higher ammonification than nitrification rates [43] , the low pH also greatly increases Fe solubility [44] . This close relationship between NH 4 + and Fe in both plants and soils should be considered when developing agronomic strategies or genetically manipulated plants to cope with NH 4 + stress. The ferroxidase LPR2 is crucial for NH 4 + -induced Fe deposition in the phloem (Fig. 3c ). Unexpectedly, the area of LPR2 distribution in root stele is much larger than the region of phloem-specific Fe deposition. Because LPR2 mainly resides in the cell wall matrix (Fig. 2a, b ), the source of LPR2 substrate from a phloem cell-specific Fe 2+ efflux may affect the specificity of NH 4 + -induced Fe deposition in the phloem. A comprehensive map of the microarray expression profiles of root cell types showed that FPN1 is mainly expressed in phloem cells [45] . Therefore, the Fe 2+ efflux protein FPN1 may also play a role in controlling the phloem specificity of Fe deposition. Nevertheless, disruption of FPN1 in T-DNA fpn1 insertion mutants did not improve PR growth under NH 4 + stress as it did in lpr2 mutants (Supplementary Fig. 25 ), refuting the above-assumed role of FPN1. Another possible mechanism is that the allocation of photosynthesis products via phloem may allow the cell wall matrix of phloem cells and their adjacent cells to accumulate greater reductants, which favors producing Fe 2+ for LPR2-catalyzed reactions. Regardless of the origin of Fe 2+ in the cell wall matrix of phloem, the massive Fe deposition in the phloem due to NH 4 + stress closely depends on the action of LPR2. Interestingly, Fe is also a key player in remolding PR development in response to inorganic phosphate ( Pi ) deficiency, which mainly depends on the actions of LPR1 [23] , [46] , [47] , [48] , [49] , [50] . However, although the amino acid sequences of LPR1 and LPR2 are 79% identical [23] , only LPR2 remolds PR development in the presence of NH 4 + as the primary N source (Fig. 1 ). The failure to restore the NH 4 + -sensitive phenotype in lpr2 mutants by confining LPR1 expression to the LPR2 action site (Fig. 2e, f ) suggests that the enzymatic actions of LPR1 and LPR2 in plants may be differently regulated. Furthermore, the tissue distribution of LPR1 also differs from that of LPR2 (Fig. 4 and Supplementary Fig. 15 ). The above differences may explain the specificity of LPR2 in mediating NH 4 + sensitivity of PRs. Importantly, the Km value of recombinant GST-LPR2 (~17 µM Fe 2+ ; Fig. 2d ) is higher than that of LPR1 (~3 µM Fe 2+ ) [27] . This discrepancy corresponds well with the discrepancy in Fe dose requirements in regulating PR growth responses to Pi deficiency and NH 4 + stress: 2.5 µM Fe was sufficient for LPR1 to inhibit PR growth under Pi deficiency [27] , but an Fe dose of more than 10 µM was required for LPR2 to inhibit PR growth under NH 4 + stress (Fig. 3 ). Fe is a co-factor for several ROS-producing enzymes, such as NADPH oxidases, cytochrome P450 enzymes, lipoxygenases, and xanthine oxidase [51] . Fe redox cycling is also capable of generating ROS directly via Fenton reactions [52] . Therefore, aberrant accumulation of Fe often triggers direct and indirect bursts in ROS [53] . Regardless of the means of Fe regulation of ROS generation, our study showed a clear burst in ROS in root phloem as a result of NH 4 + -induced Fe deposition (Fig. 5c–e ). However, we were unable to distinguish whether this burst was generated in the intra- or extracellular matrix of phloem. Considering the apoplastic Fe deposition in the phloem, the NH 4 + -induced burst of ROS is most likely an extracellular process. Studies have revealed a strong connection between callose deposition and bursts of ROS in response to external biotic and abiotic cues [33] . The ROS burst is also responsible for the induction of callose deposition in response to NH 4 + stress (Fig. 6d ). The Pi deficiency-induced PR growth inhibition was identified to be associated with enhanced callose accumulations in the elongation zone and SCN, which mainly depends on LPR1-mediated Fe deposition [26] , [47] . Unexpectedly, our study showed that although Fe deposition was also observed in the SCN in all treatments, particularly under Fe low conditions, the callose in this region did not accumulate correspondingly across the treatments (Figs. 3c and 6a ). Callose is degraded by β-1,3-glucanases [54] . Bioinformatic analyses have identified approximately 50 β-1,3-glucanase-related genes in Arabidopsis [55] . A recent single-cell RNA-Seq showed that several β-1,3-glucanase-related genes, such as At1g66250 , At2g05790 , At2g01630 ( PdBG2 ), At4g29360 , At5g42100 , and At5g58090 , are preferentially expressed in root SCN [56] . The impacts of these β-1,3-glucanases in callose accumulation in the SCN may vary in different treatments. The phloem is implicated as an important mediator of plant growth plasticity in response to environmental cues [57] . Under normal growth conditions, callose is present in the sieve plates and plasmodesmata neck region of phloem at a basal level. Heavy deposition of callose in the phloem may plug sieve pores and decrease plasmodesmal permeability [54] , [58] . Indeed, our phloem-mobile probe test using esculin provides direct evidence that NH 4 + -induced callose deposition significantly inhibits phloem transport and unloading. Sucrose is the major transport sugar in the phloem from cotyledon or mature leaves to roots, while root growth depends highly on the sucrose imported from shoot parts [57] . Esculin is loaded into the phloem in a strict sucrose transporter-dependent manner [35] , [38] . Therefore, the NH 4 + -induced inhibition of phloem action, as indicated by esculin (Fig. 7a, b ), suggests that the sucrose supply to the root growth zone may be insufficient for sustaining normal cell division and differentiation. This idea is supported by the finding that elevation of sucrose supplementation in the upper part of detached roots completely rescued PR growth under NH 4 + stress (Fig. 7c ). Previously, several physiological issues, including depletion of the carbon supply, deficiency of mineral cations (i.e., K + ), excess root energy demands associated with NH 4 + assimilation, and high energetic cost due to futile transmembrane NH 4 + cycling, were proposed as toxic actions of NH 4 + [1] , [59] . However, these actions may be related to the inhibition of sucrose transport in the phloem due to aberrant Fe deposition. This is because insufficient sucrose supply would not only directly lead to carbon depletion but also result in failure to meet the energy demands for either excess NH 4 + assimilation or futile transmembrane NH 4 + cycling. In addition, the sucrose loading into phloem requires the action of K + loading [60] , and thus a deficiency of K + caused by NH 4 + stress could further result in inhibition of sucrose transport in the phloem. Within these contexts, inhibition of phloem action as a consequence of Fe deposition could be a primary mechanism that connects the inhibition of root development to NH 4 + stress. It is worth noting that, in addition to transporting sugar, phloem also delivers other numerous substances, including proteins, RNAs, and peptides, but currently, only a few have been confirmed to be associated with a function [61] . Recently, the movement of 5-methylcytosine-modified AtTCTP1 mRNA in the phloem was shown to slightly promote PR growth of Arabidopsis [62] . In addition, the protophloem has been proposed as a nexus that senses CLE peptides that convey environmental conditions and adjusts root growth accordingly [63] . 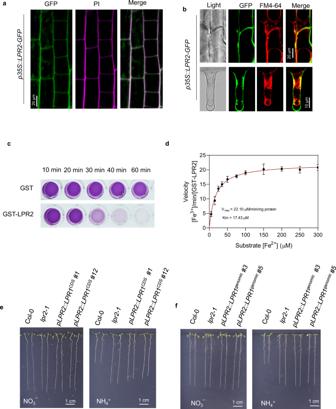Fig. 2: LPR2 is a cell wall ferroxidase and is irreplaceable by LPR1. aFluorescence co-localization of LPR2-GFP and propidium iodide in cells ofp35S::LPR2-GFProots.bFluorescence of LPR2-GFP and FM4-64 in cells ofp35S::LPR2-GFProots after plasmolysis with 0.8 M sorbitol. Four-day-old seedlings were transferred to NH4+medium with 100 µM Fe, and confocal analyses were performed 4 days after seedling transfer.cFerroxidase activities of recombinant GST-LPR2. Ferroxidase assay using 1 μg purified GST-LPR2 protein. Pink indicates the Fe2+-ferrozine complex. The substrate Fe2+was added in the form of Fe(NH4)2(SO4)2·6H2O at an initial concentration of 50 μM.dFe2+concentration-dependent (0–300 μM) ferroxidase activity of GST-LPR2 protein. Data shown are mean ± SD of three biological replicates.e,fPhenotype oflpr2-1mutant lines with LPR2 promoter-confined tissue-specific expression ofLPR1CDSandLPR1genomic. Four-day-old seedlings of the indicated genotypes were transferred to NO3−or NH4+medium with 100 µM Fe and analyzed 4 days after seedling transfer. Two (c,d) or three (a,b,e,f) independent experiments were performed with similar results, and one representative experiment is shown. In these contexts, the action of phloem in regulating PR growth is not merely limited to the movement of sucrose. Therefore, the roles of other substances, particularly signal molecules, in the regulation of PR growth inhibition from a resulting impairment of phloem action under NH 4 + stress might merit further study. In conclusion, we propose a mechanism by which root development is remolded in response to a variation in the predominant N source (Fig. 8 ). In comparison with NO 3 − as the major N source, NH 4 + induces excessive Fe deposits in the apoplast of root phloem via the action of cell wall-localized ferroxidase LPR2, which catalyzes the oxidation of Fe 2+ into Fe 3+ . Such an aberrant Fe accumulation triggers ROS generation and consequently leads to massive callose deposition. This impairs phloem action and arrests root development because of insufficient sucrose allocation to the root growth zone. Our findings may provide a strategy for improving plant adaptation to NH 4 + -rich soil environments via biotechnological pathways to manipulate Fe deposition in root phloem. Fig. 8: Schematic model of the mechanism that connects remodeling of root development to NH4+ as the primary N source. In comparison with NO 3 − as the primary N source, NH 4 + supplementation as the predominant N source induces excessive Fe deposits in the apoplast of root phloem via a catalytic reaction of Fe 2+ oxidation to Fe 3+ , which depends on the action of the cell wall-localized ferroxidase LPR2 in root stele. Such an aberrant Fe accumulation then inhibits phloem transport and unloading by triggering a burst of reactive oxygen species, which subsequently induces massive callose deposition. Consequently, sucrose is insufficiently allocated to the root growth zone, which arrests root development. Full size image Plant lines and growth conditions Wild-type A. thaliana accession Columbia (Col-0) was used as a control for all experiments. The T-DNA insertion lines lpr2-1 (SALK_091930), isas (SALK_056696), and fpn1 (SALK_055499) were obtained from the Arabidopsis Biological Resource Center (Ohio State University, Columbus, OH, USA). The lpr1-1 and lpr1-1lpr2-1 ( lpr1lpr2 ) mutants were provided by Prof Liu Dong (Tsinghua University, Beijing, China); pSUC2::GFP-sporamin and roGFP2-orp1 were provided by Prof Chun-Ming Liu (Chinese Academy of Sciences, Beijing, China) and Dr Markus Schwarzländer (University of Münster, Münster, Germany), respectively. Homozygous lines were used in this study, and the insertions were verified using the primers listed in Supplementary Data 2 . The plants were grown on a basic agar medium in sterile Petri dishes. Briefly, the seeds were surface-sterilized using 25% NaClO and sown on basal medium containing 1% (w/v) sucrose, 0.8% (w/v) agar, and MES. The nutrient composition of the basal medium was as follows: 3 mM KNO 3 , 0.5 mM (NH 4 ) 2 SO 4 , 1 mM CaCl 2 , 500 μM NaH 2 PO 4 , 500 μM MgSO 4 , 100 μM Fe(II)-EDTA, 10 μM H 3 BO 3 , 0.5 μM ZnSO 4 , 0.5 μM MnSO 4 , 0.1 μM (NH 4 ) 6 Mo 7 O 24 , and 0.1 μM CuSO 4 (pH 5.7). After vernalization at 4 °C for 2 days, the Petri dishes were moved to a controlled-environment growth chamber with a 12 h light/12 h dark cycle at 22 °C. The 4-day-old seedlings were then transferred to basic agar media with 2.5 mM (NH 4 ) 2 SO 4 or 5 mM KNO 3 as the sole N source, containing various doses of Fe(II)-EDTA as indicated in the figure legends. The resulting differences in K concentrations were balanced by adjusting the KCl concentration. To avoid a possible artificial impact from light irradiation on roots, the roots of seedlings were covered with a sterile black plastic sheet, as depicted in Supplementary Fig. 3a . Generation of transgenic plants For the generation of plant expression vectors for genetic complementation, the 5949-bp genomic DNA of LPR2 (including a 2928-bp region upstream of the start codon) and the 4262-bp genomic DNA of LPR1 (including a 2178-bp region upstream of the start codon) were cloned into a pEarleyGate 101 vector containing a YFP reporter. The resulting constructs pLPR2::LPR2-YFP and pLPR1::LPR1-YFP were then transformed into lpr2-1 and lpr1-1 mutants, respectively, to generate complementation lines ( pLPR2::LPR2-YFP / lpr2-1 and pLPR1::LPR1-YFP / lpr1-1 , respectively). For analysis of subcellular localization of LPR2, the LPR2 coding sequence (CDS), fused to GFP, was cloned into a modified pCAMBIA1300 vector containing a doubled CaMV 35S promoter. The resulting construct was transformed into Col-0 to obtain the p35S::LPR2-GFP line. For the LPR2 promoter-confined complementation assay of LPR1 , the 2928-bp region upstream of the start codon of LPR2 , together with either the CDS or genomic sequence of LPR1 , was cloned into a pCAMBIA1300 vector. The resulting construct was transformed into lpr2-1 mutants to generate pLPR2::LPR1 CDS / lpr2-1 or pLPR2::LPR1 genomic / lpr2-1 transformants. All primers used for vector construction are listed in Supplementary Data 2 . All transgenic lines were generated by agrobacterium-mediated transformation using the floral dip method. Only homozygous lines were used in this study. Measurements of root meristem size and cell elongation Measurements of root meristem size and cell elongation were performed 4 days after seedling transfer to the indicated media. The roots were incubated in 10 μg mL –1 propidium iodide (PI; Sigma-Aldrich, St. Louis, MO, USA) in the dark for 5 min and rinsed twice with deionized water. The roots were then imaged by confocal microscopy. Root meristem size was measured as the number of cortical cells between the quiescent center and the first elongated cell (Supplementary Fig. 3b ). The average number of elongating cells in the same cell file was calculated from the first elongating cell to the first differentiating cell. The length of the latter cell type was measured to calculate the average length of the first differentiating cells. Histochemical Fe staining The histochemical Fe staining of roots was adapted from the method of Roschzttardtz et al. [22] . Briefly, after 4 days of treatments in the indicated media, the roots were incubated for 45 min under vacuum (500 mbar) with Perls’ staining solution (2% [v/v] HCl and 2% [w/v] potassium ferrocyanide). After being rinsed three times with deionized water, the root samples were incubated for 1 h in a methanol solution containing 10 mM NaN 3 and 0.3% H 2 O 2 . Subsequently, the root samples were washed with 100 mM Na-phosphate buffer (pH 7.4) and intensified by 5 min incubation in the same buffer containing 0.025% (w/v) DAB and 0.005% (v/v) H 2 O 2 . The reaction was stopped by washing with deionized water and optically cleared with chloral hydrate. Stained root samples were observed using a differential interference contrast microscope (Nikon, Tokyo, Japan). Confocal microscopy and staining procedures Confocal analyses were performed on either an Olympus FV3000 (Tokyo, Japan) or a Zeiss LSM 880 microscope (Oberkochen, Germany). For callose staining, roots were incubated in 150 mM K 2 HPO 4 and 0.01% (w/v) aniline blue in the dark for 2 h. For ROS staining, roots were incubated with 10 μM H 2 DCFDA (Beyotime Biotech, Shanghai, China) in the dark for 30 min and then washed twice with deionized water. For PI or FM4-64 staining, roots were directly imaged in 10 μM PI or 4 μM FM4-64 (Thermo Fisher Scientific, Waltham, MA, USA). The excitation (ex)/emission (em) parameters for confocal analyses are as follows: GFP/YFP/H 2 CDFA ex: 488 nm, em: 500–550 nm; PI/FM4-64 ex: 561, em: 570–670 nm; aniline blue ex: 405 nm, em: 475–525 nm; esculin ex: 405 nm, em: 420–480 nm; and roGFP2-Orp1 ex: 405 and 488 nm in sequence, em: 505–535 nm and 425–475 nm (auto fluorescence recorded at ex: 405 nm for subtraction in calculating the ratio 405/488 nm) [29] . Analysis of esculin movement The esculin movement in the phloem of PRs was detected as described by Knox [36] . Briefly, after 4-day treatment with the indicated media, cotyledons were pretreated with 0.3 μL 2.5% (v/v) Adigor solution (Syngenta, Basel, Switzerland) for 1 h and subsequently supplemented with 0.5 μL 9 mg mL –1 esculin solution. After 10 min, the appearance of esculin in the phloem of the PR was noted. Then, the fluorescent front in root phloem was marked on the plate, and the time was noted. Thereafter, the fluorescence in root phloem was re-checked after 10 min, and the new front was marked along with the time. The distance of esculin movement in the phloem was taken as the length between the two marks. The PTV was calculated from the distance and the interval time. In addition, once esculin was imported into the root tip, individual images, with their times of acquisition, were recorded to evaluate the unloading of the phloem unloading [37] . In vitro ferroxidase characterization of recombinant proteins The LPR2 CDS without signal peptide sequences were cloned into pGEX-6P-1, which enables the fusion of a GST tag. Isopropyl β-D-1 thiogalactopyranoside (0.5 mM) was supplied to Escherichia coli strain Arctic Express carrying pGEX-6P-1 or pGEX-6P-1-LPR2 at 14 °C for 20 h to induce expression of the GST or GST-LPR2. The cells were harvested by centrifugation (4000 × g , 30 min, 4 °C) and lysed in extraction buffer (50 mM Tris-HCl (pH 7.4), 150 mM NaCl, 1 mM PMSF, and 100 μg·mL −1 mL lysozyme) with sonication. After centrifugation at 15,000 × g at 4 °C for 30 min, the supernatant was recovered, then the GST or GST-LPR2 protein was purified using a column containing Glutathione Sepharose 4B beads (Solarbio, Beijing, China) [64] . The purified proteins were further desalted and concentrated using centrifugal filter (Merck Millipore, Amicon Ultra 15, molecular weight cut-off of 10 kDa). Ferroxidase activity was measured using a ferrozine-based method [26] . Briefly, a defined amount of protein was mixed with various amounts of ferrous ammonium sulfate in a solution of 0.1 M sodium acetate with 100 μM CuSO 4 (pH 5.0) to reach desired substrate concentrations. After incubation, 200-μL samples were taken in appropriate intervals and transferred to 96-well plates for reaction-quenching with 14 μL 18 mM ferrozine. The absorbance at 560 nm was measured using a plate reader (SpectraMax i3x; Molecular Devices, San Jose, CA, USA). The decrease in the substrate was then used to calculate the oxidation of Fe 2+ . The K m and V max were calculated using the Michaelis–Monod model in GraphPad Prism 8 software (GraphPad Software, San Diego, CA, USA). Determination of ammonium Root samples were ground in liquid N 2 immediately after collection. One milliliter of 0.3 mM sulfuric acid solution was added to the frozen powder, followed by vortexing. The mixture was centrifuged at 12,000 × g at 4 °C for 10 min. The NH 4 + concentration in the supernatant was determined colorimetrically using a method based on the phenol-hypochlorite assay at 635 nm in a spectrophotometer [10] . Quantitative real-time RT–PCR After 4-day treatment in the indicated media, the total RNA in roots was extracted using RNAisoPlus (Takara, Kyoto, Japan) and treated with DNase I to remove contaminant genomic DNA. We synthesized cDNA using a PrimeScript RT reagent kit (Takara) according to the manufacturer’s protocol. 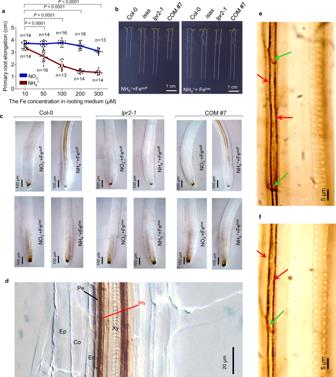Fig. 3: Fe-dependent inhibition of primary root growth in NH4+ medium. aPrimary root elongation of Col-0 seedlings in NO3−-N or NH4+-N source with various doses of Fe. Center line represents mean and bounds of box are SD; whiskers indicate the minimum and maximum values;n= number of seedlings.Pvalues <0.05 indicate significant interactions between N form and Fe dose (two-way ANOVA with post-hoc Tukey HSD test).bNH4+-sensitivity comparison of Col-0,isas,lpr2-1, and complementation line COM#7 in Fesuff(100 µM) and Felow(10 µM) conditions.cFe deposition indicated by Perls/DAB staining in primary roots.dClose-up view of Fe deposition in root stele of Col-0 seedlings grown in FesuffNH4+medium. Ep epidermis, Co cortex, En endodermis, Pe pericycle, Ph phloem, Xy xylem.ePerls/DAB staining in the phloem of the primary roots of Col-0 seedlings grown in FesuffNH4+medium. Red and green arrows show Fe depositions at lateral cell walls and sieve plates of the phloem, respectively.fAcetone washed-Perls/DAB staining in phloem of the primary roots of Col-0 seedlings grown in FesuffNH4+medium. The Perls/DAB-stained roots were washed with acetone for 3 h. Four-day-old seedlings of the indicated genotypes were transferred to NO3−or NH4+medium with various doses of Fe supply and analyzed 4 days after seedling transfer. Each experiment was repeated independently three times with similar results, and a representative experiment is shown. We performed qRT-PCR analysis of LPR2 with TB Green Premix Ex Taq II (Takara) on a Step One system (Agilent Technologies, Santa Clara, CA, USA). The primers used for qRT-PCR analysis are listed in Supplementary Data 2 . UBQ10 and EF1α were used as the reference genes. Relative transcript abundances were determined by normalizing to the geometric mean of expression of two reference genes for each sample [65] . Immunoblot analysis Polyclonal LPR2 epitope-specific antibody was raised in rabbits against a synthetic peptide (LPR2:DEGGIKQEERLFNLGKLE-C) and affinity-purified (ABclonal, Wuhan, China). After 4-day treatment in the indicated media, the total root proteins were extracted using a Plant Protein Extraction Kit (Solarbio, Beijing, China) following the manufacturer’s protocol. The protein samples were separated in 10% SDS/PAGE gels and transferred to nitrocellulose membranes (Bio-Rad, Hercules, CA, USA) in semi-dry conditions (Trans-Blot SD semi-dry transfer cell; Bio-Rad). The membranes were incubated in blocking buffer (TBST, 5% milk powder) at room temperature for 2 h and then incubated overnight in blocking buffer containing anti-LPR2 antibody (1:2000), rabbit polyclonal anti-GFP (1:5000; catalogue no. AE011, ABclonal, Wuhan, China) or mouse monoclonal anti-actin antibody (1:2000; catalogue no. D191048, Sangon Biotech, Shanghai, China) at 4 °C. HRP-conjugated goat anti-rabbit IgG (1:5000; catalogue no. D110058, Sangon Biotech) or goat anti-mouse IgG (1:5000, catalogue no. D110087, Sangon Biotech) was used as a secondary antibody. The signal was detected using an ECL Kit (Tanon™; AbClon). In addition, the membranes were also stained with Ponceau S to visualize total proteins as the loading reference. RNA sequencing and GO analysis After 4-day treatment in the indicated media, the total RNA was extracted from the roots of Col-0 and lpr2-1 seedlings using MagZol Reagent (Magen, Guangzhou, China) following the manufacturer’s protocol. We constructed mRNA-Seq libraries using NEBNext Ultra RNA Library Prep Kit for Illumina (NEB, Ipswich, MA, USA). The quality of the libraries was assessed using an Agilent 2100 Bioanalyzer. Sequencing was performed using a Hiseq Xten sequencer (Illumina, San Diego, CA, USA) at RIBOBIO (Guangzhou, China). Raw reads were quality controlled and trimmed using FastQC v0.11.8 ( http://www.bioinformatics.babraham.ac.uk/projects/fastqc/ ) and Trimmomatic. 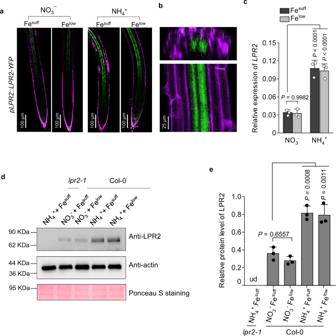Fig. 4: Distribution of LPR2 in roots and its response to NH4+. apLPR2::LPR2-YFPexpression in primary roots of complementation line COM#7. Roots were counterstained with propidium iodide (purple fluorescence) and analyzed for YFP fluorescence (green).bRadial section (top) and close-up view (bottom) ofpLPR2::LPR2-YFPexpression in a root of a COM#7 seedling grown in FesuffNH4+medium.cLPR2expression in Col-0 roots. Relative expression levels were normalized to the geometric mean of expression ofUBQ10andEF1α.d,eRepresentative gels and relative protein levels in Col-0 roots. Relative LPR2 levels were estimated from the ratio of the signal intensity of LPR2 to that of actin from the same sample.c,eData shown are mean ± SD of three biological replicates.Pvalues < 0.05 indicate significant differences (two-way ANOVA with post-hoc Tukey HSD test). Four-day-old seedlings of the indicated genotypes were transferred to NO3−or NH4+medium with Fesuff(100 µM) or Felow(10 µM) and analyzed 4 days after seedling transfer. Each experiment was repeated independently three times with similar results, and a representative experiment is shown. The clean reads were mapped to the Arabidopsis genome (TAIR10) using HISAT2 and a GTF annotation file from the Ensembl Plants database ( ftp://ftp.ensemblgenomes.org ) and then analyzed using Stringtie and ballgown [66] . 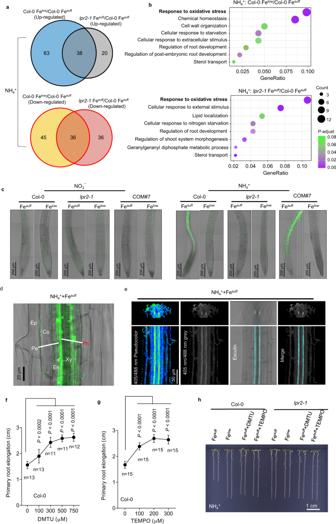Fig. 5: Fe-dependent primary root growth inhibition by NH4+ is associated with a burst in reactive oxygen species (ROS). a,bVenn diagram and Gene Ontology enrichment analysis of differentially expressed genes (DEGs) that are up- and downregulated in the pairwise comparisons of Col-0 Felowvs. Col-0 Fesuffandlpr2-1Fesuffvs. Col-0 Fesuffin the NH4+-N source. The size of the circle represents gene numbers, and the color represents the value ofP-adjust the was calculated by hypergeometric tests and adjusted for multiple testing using FDR. RNA sequencing was conducted with three biological replicates per line and condition.cROS visualization in primary roots of Col-0,lpr2-1, and complementation line COM#7 seedlings by H2DCFDA staining.dClose-up view of H2DCFDA staining in primary roots of Col-0 seedlings grown in FesuffNH4+medium.eCo-localization of false color representation of H2O2and fluorescence of phloem marker esculin in primary roots of roGFP2-Orp1 seedlings grown in FesuffNH4+medium.f,gDose-response relationship of the primary root elongation of Col-0 seedlings plotted as a function of the concentration of ROS scavengers. Data shown are mean ± SD.n= number of seedlings.Pvalues < 0.05 indicate significant differences (one-way ANOVA with post-hoc Tukey HSD test).hImages of the effects of 750 µM dimethyl thiourea (DMTU) and 200 µM 4-hydroxy-TEMPO (TEMPO) on Col-0 seedlings. Four-day-old seedlings of the indicated genotypes were transferred to NO3−or NH4+medium with Fesuff(100 µM) or Felow(10 µM) with or without the indicated ROS scavengers. Analyses were performed 4 days after seedling transfer. The experiments (c–h) were repeated independently three times with similar results, and representative data from one experiment are shown. Significant DEGs were assessed using a P value threshold of <0.05 and |log 2 (fold change)| > 1 using DEGseq [67] . 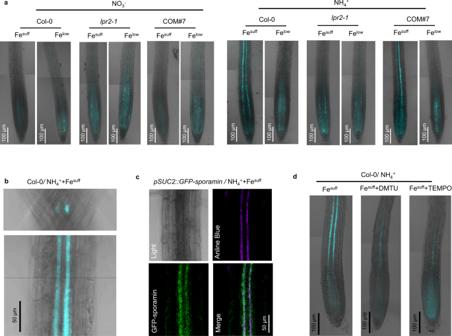Fig. 6: Fe-dependent callose deposition in the phloem via reactive oxygen species (ROS) in response to NH4+. aCallose detection in primary roots of Col-0,lpr2-1, and complementation line COM#7 seedlings by aniline blue staining.bRadial section (top) and close-up view (bottom) of aniline blue staining in primary roots of Col-0 seedlings grown in FesuffNH4+medium.cFluorescence co-localization of GFP-sporamin and aniline blue staining inpSUC2::GFP-sporaminroots.dROS scavengers abolished the NH4+-induced callose deposition. Four-day-old seedlings of the indicated genotypes were transferred to NO3−or NH4+medium with Fesuff(100 µM) or Felow(10 µM) with or without the indicated ROS scavenger. Each experiment was repeated independently three times with similar results, and a representative experiment is shown. GO term enrichment analysis was performed with R packages clusterProfiler and database org.At.tair.db (version 3.13.0) [68] . Statistical analyses Data were analyzed by one-way and two-way ANOVA with post-hoc Tukey HSD test using Prism v8 (GraphPad). A P value < 0.05 was considered statistically significant. 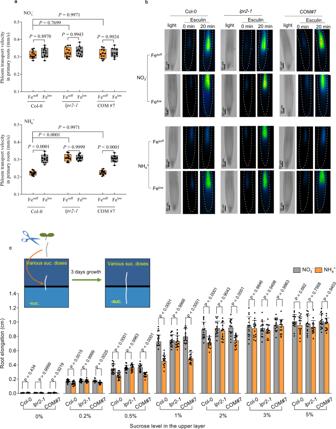Fig. 7: Inhibition of phloem action and sucrose complementation of primary root growth in NH4+ medium. a,bPhloem transport velocity and phloem unloading of esculin. Center line represents mean and bounds of box are SD; whiskers indicate the minimum and maximum values.Pvalues < 0.05 indicate significant differences (two-way ANOVA with post-hoc Tukey HSD test,n= 12 seedlings per line and condition). Four-day-old seedlings of Col-0,lpr2-1, and complementation line COM#7 were transferred to NO3−or NH4+medium with Fesuff(100 µM) or Felow(10 µM) and analyzed 4 days after seedling transfer.cGrowth response of detached primary roots to localized sucrose supply. Data shown are mean ± SD.Pvalues < 0.05 indicate significant differences (two-way ANOVA with post-hoc Tukey HSD test,n= 16 detached primary roots per line and condition). Inset: Scheme depicting the growth response analyses of detached primary roots to localized sucrose supply. Roots (1 cm) were cut from four-day-old seedlings. The detached roots were then transferred to a vertical two-layer split agar system of either NO3−or NH4+medium with Fesuffor Felow. The upper layers were treated with various doses of sucrose, and the lower layers were absent of sucrose. Analyses were performed 3 days after seedling transfer. Each experiment was repeated independently three times similar results, and a representative experiment is shown. 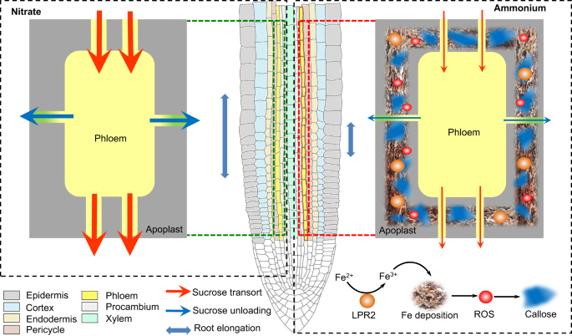Fig. 8: Schematic model of the mechanism that connects remodeling of root development to NH4+ as the primary N source. In comparison with NO3−as the primary N source, NH4+supplementation as the predominant N source induces excessive Fe deposits in the apoplast of root phloem via a catalytic reaction of Fe2+oxidation to Fe3+, which depends on the action of the cell wall-localized ferroxidase LPR2 in root stele. Such an aberrant Fe accumulation then inhibits phloem transport and unloading by triggering a burst of reactive oxygen species, which subsequently induces massive callose deposition. Consequently, sucrose is insufficiently allocated to the root growth zone, which arrests root development. Reporting summary Further information on research design is available in the Nature Research Reporting Summary linked to this article.